Spread of white-nose syndrome on a network regulated by geography and climate Wildlife and plant diseases can reduce biodiversity, disrupt ecosystem services and threaten human health. Emerging pathogens have displayed a variety of spatial spread patterns due to differences in host ecology, including diffusive spread from an epicentre (West Nile virus), jump dispersal on a network (foot-and-mouth disease), or a combination of these (Sudden oak death). White-nose syndrome is a highly pathogenic infectious disease of bats currently spreading across North America. Understanding how bat ecology influences this spread is crucial to management of infected and vulnerable populations. Here we show that white-nose syndrome spread is not diffusive but rather mediated by patchily distributed habitat and large-scale gradients in winter climate. Simulations predict rapid expansion and infection of most counties with caves in the contiguous United States by winter 2105–2106. Our findings show the unique pattern of white-nose syndrome spread corresponds to ecological traits of the host and suggest hypotheses for transmission mechanisms acting at the local scale. Wildlife and plant diseases can reduce biodiversity, disrupt ecosystem services and threaten human health [1] , [2] , [3] . White-nose syndrome (WNS), a highly pathogenic infectious disease caused by the cryophilic fungus Geomyces destructans , has emerged in North American Vespertilionid bats, and is currently spreading [4] , [5] , [6] , [7] throughout the Eastern United States and Canada. WNS was first observed in 2006 in Schoharie County, NY, and within 2 years spread to 15 counties within a ∼ 230 km radius [4] . The speed of this spread, together with early reports of mass mortality in infected caves, has generated concern about massive depletion of currently common bat species, attendant loss of economic services, and transmission to vulnerable populations of threatened and endangered species [5] , [8] , [9] , [10] . Although WNS has now been reported in 20 states and up to ∼ 2,220 km from its North American origin, the ecological and environmental determinants of these epidemiological dynamics are poorly understood. Understanding the mechanisms by which WNS will expand is crucial to management of infected and vulnerable bat populations and the conservation of threatened and endangered bat species. Particularly important is determining where and how fast WNS will spread. Historically, emerging pathogens have displayed a variety of spatial spread patterns due to differences in host ecology, including diffusive spread from an epicentre (West Nile virus [11] ), stratified diffusion (rabies virus [12] ), jump dispersal on a network (foot-and-mouth disease virus [13] ) or a combination of these ( Phytophthora ramorum [14] ). Diffusive spread is expected for pathogens with highly mobile host species (for example, migratory passerines that transport West Nile virus), while jump dispersal is expected for patchily distributed species with unequal time scales of within- and between-patch transmission (for example, livestock farms that mediated foot-and-mouth disease). Either of these patterns is consistent with the natural history of bats: cave-dwelling bats exhibit long-distance aerial migration [15] and high levels of seasonal mixing [16] , [17] , but bats in temperate North America are also associated with patchily distributed geologic formations, particularly karst outcrops of the Appalachian range and Interior Plateaus and Highlands [18] . How WNS should be expected to spread is, therefore, an open question. To determine which of these two scenarios predominates in the spatial spread of WNS, we used maximum likelihood (ML) estimation to fit a series of models to data on the county-scale infection history of this epidemic. We started with a simple diffusion model and added complexity to create spatially structured networks and then complex heterogeneous networks where patches differed in attributes. We hypothesized that: geographic complexity gives rise to corridors that facilitate spread along the dominant cave-bearing geologic formations, spread is accelerated by high concentrations of caves, and spread is retarded in warmer areas due to the shorter duration of cold temperatures through direct and indirect influences on bat condition and fungal growth. We tested these hypotheses through statistical comparison of alternative models where the probability that county i does not become infected from previously infected county j had the general form: The function f describes the inverse of transmission intensity from j to i , numerically representing alternative hypotheses about the determinants of transmission. To further examine possible scenarios, we fit additional models of moderate complexity, as well as an epidemiological model [19] and a complex radiation model [20] . The radiation model used the same general form as above, but the epidemiological model directly calculated . Simulations forward in time allowed us to compare spatial characteristics and predict future scenarios of spread under assumptions of our best-supported model. We found the best fit model was of moderate complexity and included covariates regarding the number of potential hibernacula and length of winter. Simulations forward in time based on this model suggest that spread to counties with caves will peak by 2015–2016 in the contiguous United States. While climate change may negatively impact spread to uninfected counties according to interpretation of coefficients, applying the model to currently available projections of scenarios did not slow spread or further restrict the geographic expansion. This study suggests that a variety of hibernating bat species are at risk and that populations across the contiguous United States eventually may be exposed. Observed characteristics of spread Inspection of summary statistics of observed data indicated that spread was variable over space and time in terms of four metrics (number of counties newly infected, maximum distance of infected counties from the origin, median distance of infected counties from the origin, and area of the convex hull of infected counties, Supplementary Table S1 ). Particularly, the highest number of new WNS infections and farthest spread occurred in the fourth epidemic winter and most newly infected counties (89%) have been relatively close (<500 km) to older infections, suggesting extremely long distance dispersal events are rare ( Supplementary Fig. S1 ). Comparison of dispersal model fits Using parameters determined through ML estimation, predicted disease spread better matched observed data and was faster when diffusion models were restricted by geographic complexity (that is, to counties with caves) as opposed to diffusion over all counties ( Supplementary Fig. S2–S5 , Supplementary Table S2 ). However, there was even greater support for models that also accounted for heterogeneity in habitat and climate. 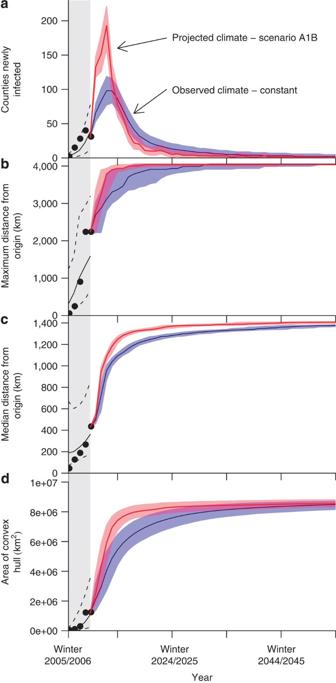Figure 1: Spread statistics for WNS based on gravitycaves+winter model ML parameter set. Gray shading represents simulated spread from Schoharie County, New York to the present and unshaded represents forecasts obtained by forward simulation from the current (2010–2011) state. Simulations forward were based on climate remaining as observed during the epidemic (blue) or as projected under the SRES A1B climate scenario (red), which tended to have longer winters (Supplementary Information). Solid lines are median values and dotted lines/shaded areas represent 95% prediction intervals. (a) The number of newly infected counties in the given winter; spread peaks in the winter of 2013–2014, and infection rate is consistent with observations in the first 5 winters of spread. (b,c) The maximum (b) and median (c) distance from Schoharie County; maximum distance from the origin will not be complete until the winter of 2032–2033. (d) The convex hull of infection area is the total area within the minimum convex polygon of infected county centroids. A generalized gravity model, which included pairwise interactions among counties based on distance and density of caves in each county (a proxy for the distribution of available hibernacula), had higher support (Akaike Information Criterion, AIC gravity _caves =760; Table 1 ) than two diffusive spread models constrained to counties with caves (AIC simple =794, AIC long-distance =774) and a similar model using county area as the gravitational mass variable (AIC gravity_area =782); the additional term in gravity models explained a significantly greater fraction of variation in the observed data than the simple diffusion model ( Table 1 , Supplementary Table S3 ). Adding winter length as an additional covariate further improved the model fit (AIC gravity_caves+winter =702). A comparison with an alternative model in which geographic position was substituted for winter length confirmed that this effect is due to climate (AIC gravity_caves+northing =728), not latitude. Bat species richness did not improve model fit over the gravity caves +winter model (AIC gravity_caves+species-richness =730, AIC gravity_caves+hibernating =740 AIC gravity_caves+winter+species-richness =702). Likewise, the epidmeological and the radiation model categorically fit less well than the gravity caves +winter model (AIC force of infection =710, AIC radiation =776) Table 1 ML parameters* for the eleven models of spread and goodness of fit to the observed data. Full size table Simulations of the best-supported model (gravity caves +winter) effectively captured each of the measured spatial features of spread ( Fig. 1 ). Empirical observations of our summary statistics were all within 95% prediction intervals generated by the simulations ( Fig. 1 ). Further, the year of known infection of specific counties was within 95% of simulations in 106 of 112 (94.6%) infected counties ( Fig. 2 ). Parameters drawn to estimate sampling uncertainty (SU) yielded similar mean values of all quantities with larger prediction intervals corresponding to the combined effects of stochastic variation and parameter uncertainty ( Supplementary Figs S6, S7 ; 107 of 112 counties within confidence bounds). By contrast, under ML parameters, all other models underestimated the observed infection rate (number of new counties infected each winter), although matches between area and distance measures for these models and observed data were typically satisfactory ( Supplementary Figs S8–S13 ). Observed year of infection generally was earlier than predicted and outside prediction intervals for the simple diffusion and simple diffusion with long-distance dispersal models, and while gravity caves and gravity caves +northing models performed better than diffusion models, they did not outperform the gravity caves +winter model ( Supplementary Figs S2–S5, S14, S15 ). Simulations using SU parameters were consistent with these observations ( Supplementary Figs S16–S27 ). In conclusion, we found the gravity caves +winter model to be the best fit overall (lowest AIC) and the only model consistent with large-scale measurements of spread. Figure 1: Spread statistics for WNS based on gravity caves +winter model ML parameter set. Gray shading represents simulated spread from Schoharie County, New York to the present and unshaded represents forecasts obtained by forward simulation from the current (2010–2011) state. Simulations forward were based on climate remaining as observed during the epidemic (blue) or as projected under the SRES A1B climate scenario (red), which tended to have longer winters ( Supplementary Information ). Solid lines are median values and dotted lines/shaded areas represent 95% prediction intervals. ( a ) The number of newly infected counties in the given winter; spread peaks in the winter of 2013–2014, and infection rate is consistent with observations in the first 5 winters of spread. ( b , c ) The maximum ( b ) and median ( c ) distance from Schoharie County; maximum distance from the origin will not be complete until the winter of 2032–2033. ( d ) The convex hull of infection area is the total area within the minimum convex polygon of infected county centroids. 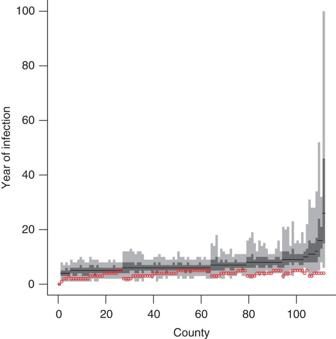Figure 2: Predicted year of infection for currently infected counties based on gravitycaves+winter model and ML parameter set. The predicted year of infection for the currently (2010–2011) infected counties based on simulations from Schoharie County using the gravitycaves+winter model and ML parameter set. For each county, the 95% prediction interval is in gray with the interquartile range specified by dark gray and the simulated mean infection year as a black bar; red dots represent the observed year of infection for that county. Counties are ordered by the simulated year of infection. Observations are generally within the confidence bounds (106 of 112 counties). Full size image Figure 2: Predicted year of infection for currently infected counties based on gravity caves +winter model and ML parameter set. The predicted year of infection for the currently (2010–2011) infected counties based on simulations from Schoharie County using the gravity caves +winter model and ML parameter set. For each county, the 95% prediction interval is in gray with the interquartile range specified by dark gray and the simulated mean infection year as a black bar; red dots represent the observed year of infection for that county. Counties are ordered by the simulated year of infection. Observations are generally within the confidence bounds (106 of 112 counties). Full size image Assessment of assumptions and simulations forward We tested our assumption that infection of a county was detected in its first year with further simulations. Our estimates were robust to incomplete detection, as even under high levels of missed infections (25% of infected counties go undetected) the resulting bias was minimal ( Supplementary Fig. S28 ). Imperfect detection introduced no detectable bias into most measures of spread, although high rates of under-detection occasionally resulted in slight deviations from zero for the area of the convex hull and the median distance from the origin ( Supplementary Fig. S28 ). With high levels of under-detection we found some statistically significant under-predictions of the number of new counties infected, but the magnitude of the bias was small. These results showed this slight underestimate will take place for the filling in of infected counties in the interior of the infected area, but not for the broader extent of the infection. The results of the under-sampled simulation demonstrate a similar pattern of spread to the observed data and the predicted year of infection is consistent for counties ( Supplementary Figs S29, S30 ). Specifically, under-detection led to more rapid spread into the West by no >5 years, but reduced spread was predicted into the Southeast and Southwest. For spread continuing under constraints of these initial 5 years, the gravity caves +winter model predicted the number of newly infected counties that contain caves will peak in the winter of 2013–2014 (95% prediction interval of 2013–2014 to 2014–2015). These projections suggest WNS will extend the maximum distance from the origin by 2032–2033 and will continue to fill in over the next 73 years, such that 93% (±1%) of counties with caves will be infected by the winter of 2105–2106 ( Supplementary Table S4 ). The predicted trajectory of spread is WNS will reach the Rocky Mountains in the next 5 years before moving more slowly to the west coast ( Fig. 3 ), whereas areas of high conservation concern in the Southeast and Texas are not predicted to become infected until much later. Indeed, many of these counties and those in the Southwest went uninfected for >100 years in several simulations ( Supplementary Fig. S16 ). Simulations using SU parameter sets were consistent with these results ( Supplementary Figs S31–S33 , Supplementary Table S5 ). In addition, we considered possible effects of projected climate change by using available simulations of future daily temperature. As North American winters have been relatively warm recently, these simulations predicted slightly faster spread of WNS despite the expected increase in temperature overall ( Fig. 1 , Supplementary Figs S34, S35 , Supplementary Table S6 ). However, the overall geographic characteristics of spread were consistent with the observed winter data used to fit the model, despite differences in speed ( Supplementary Figs S36–S41 ). 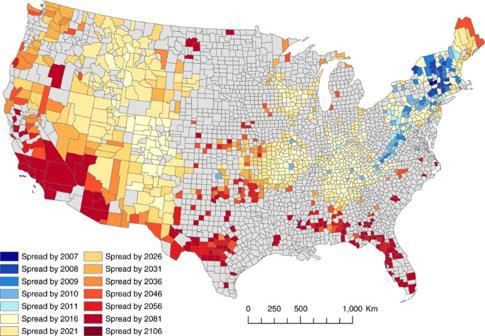Figure 3: Mean estimated year of infection under the gravitycaves+winter model using the ML parameter set. Mean estimated year of infection (yellow-to-red scale) under the gravitycaves+winter model for simulations using the ML parameter set begun from currently infected counties (2010–2011; blue colour scale). Gray counties did not have reported caves or WNS observations. The model predicts spread to most (93%±1%) of the counties with caves in the contiguous United States within a century of the first infection, many within the next 20 years. Spread to the southeast is slow as is spread to the southwest; longer time to infection in the Upper Midwest and New England may be due to edge effects (Supplementary Information). Figure 3: Mean estimated year of infection under the gravity caves +winter model using the ML parameter set. Mean estimated year of infection (yellow-to-red scale) under the gravity caves +winter model for simulations using the ML parameter set begun from currently infected counties (2010–2011; blue colour scale). Gray counties did not have reported caves or WNS observations. The model predicts spread to most (93%±1%) of the counties with caves in the contiguous United States within a century of the first infection, many within the next 20 years. Spread to the southeast is slow as is spread to the southwest; longer time to infection in the Upper Midwest and New England may be due to edge effects ( Supplementary Information ). Full size image WNS has spread from a single New York county north to Maine, south to Alabama and west to Oklahoma. Simple diffusive models are not as well supported by data from the initial 5 years of WNS spread as models that include spatial heterogeneity and a key environmental covariate, winter duration. Particularly, because a larger distance between two counties decreased the probability of infection (that is, parameter β 1 was positive for all fit models), the presence of geographic corridors due to the spatial pattern of counties with caves accelerated spread of WNS. Further, in generalized gravity models, the parameter β 2 was always positive indicating that the probability of infection increased with increasing number of caves in each county ( Table 1 ). This suggests that density-dependent transmission at higher bat population densities may facilitate spread by increasing contact rate, possibly during swarming. Furthermore, a county-level climate variable, length of winter, was an important predictor and the related parameter, β 3 , was always negative indicating increased transmission probability to colder counties ( Table 1 ). This pattern may reflect the fungus’s physiological tolerances or increased bat survival in longer summers. This result is consistent with the conclusion that WNS mortality is predictable under certain environmental conditions within Appalachia [21] . There has been a great deal of interest in the effect of species diversity on spread of multi-host pathogens. Inclusion of species richness improved performance when added to the basic gravity caves model, and the positive coefficient might be interpreted to suggest that higher values of species richness retard the spread of WNS. However, this model is equally well supported as the gravity caves +northing model, possibly reflecting the latitudinal gradient of species richness along the eastern seaboard. Further, substituting the complete bat species richness covariate with only those bats that hibernate did not improve fit to the observed data. Ultimately, species richness did not provide additional information when included with the winter covariate in a gravity model. Future studies seeking to elucidate the role of species richness in G. destructans transmission should include information about the specific regions or locations where hibernation occurs, that is, the spatial scales at which species ecological interactions may occur. Thus, overall, our model suggests that the pattern of WNS spread results from a combination of both spatially diffusive mechanisms (that is, migratory events and movement between hibernacula) and spread on a network (that is, clustering of habitats), and that there exist within- and between-region interactions that facilitate pathogen expansion. Empirical data support this conclusion as small-scale features of habitat, species occurrence and species traits can mediate the appearance within hibernacula [22] . Our modelling framework cannot account explicitly for these factors, but does not discount such factors as important mechanisms of spread. Forward simulations initialized with an infection in Schoharie County, New York captured many features of spread observed in data, but were unable to correctly predict year of infection within quartiles for some counties, consistent with other simulation studies [23] . Our goal in this study was to compare simple diffusive and geographically complex spread models that captured the characteristics of WNS expansion; the observed pattern of occurrence is one potential realization of the spread dynamics and stochastic processes make predictions for individual counties challenging and possibly ineffectual. Counties that were regularly under-predicted were those in Oklahoma and Missouri, which we consider to be possibly anomalous. Particularly, the occurrence in Oklahoma represents a single live bat that tested positive for the pathogen and the pattern of infection differed from bats from the East Coast [24] . We also note that bats readily use anthropogenic features [25] that also can be suitable habitat for G . destructans , which would facilitate spread and thus bias our predictions where our proxy for available habitat (cave density) is incomplete. However, recent analysis of WNS spread in the northeastern US suggests that mines are less likely to become infected than caves [26] , suggesting that this bias may not be as great as one might fear. Thus, counties without caves but with mines may incur infection, but that the effect of these infections on spread will probably be small. By simulating the effect of imperfect detection on model evaluation, we found that high levels of under-detection did not substantially bias summary statistics. Furthermore, it is likely that detection following the first 2 years was very high given the profile of the disease. As we considered data at the county-level using a compartmental model, not the level of the individual cave, we reduced the chance that we missed a critical data point while simultaneously removing potential issues of prevalence and within-county dynamics. Accordingly, we found our results to be very robust to probable levels of under-detection. It has been reported that the management of other emerging diseases would have benefited from earlier predictions of spread [27] . Our study sought to examine how the epidemic will progress under the constraints and assumptions of the gravity caves +winter model using ML and SU parameter sets by extrapolating from the state of infection as of 1 June 2011. These simulations provide both general properties of anticipated spread (that is, approximate time frame for invasion of biologically sensitive areas), and specific estimates (with prediction intervals) for all counties in the contiguous United States. Short-term predictions (that is, those within 10 years) are both most reliable and relevant to actions that might be taken immediately; long-term predictions (that is, those well into the future) are less certain due to demographic stochasticity and potential population collapse [9] , [10] , as well as uncertainty about future climate conditions [28] and future control measures. Our choice in simulation duration (to 2105 under stable climate and 2100 for climate change scenarios) reflects the temporal extent of available climate change forecasts, not necessarily considerations about a priori expectations of the progression of WNS epidemic. Additionally, because these predictions assume that regionally different host communities do not differentially affect spread, future spread may be different than predicted in proportion to inhomogeneity in host communities and/or the extent that resistance to infection is evolved [22] , [29] . What will happen next? Our forward simulations from the observed distribution of WNS under ML parameters predicted that infection rate of new counties will peak in the winter of 2013–2014 (+1 winter) and that WNS will reach the maximum distance from Schoharie County in the winter of 2032–2033. Under the assumption that the first 5 years of spread are indicative of the future pattern, our models predicted spread will continue rapidly along and within the Appalachians, filling in counties that were jumped over until reaching the southeast. As a result, potentially susceptible species such as the Indiana Bat ( Myotis sodalis ) and Gray Bat ( M. grisescens ) will be of concern due to their already endangered status. Spread will be slow into the western United States, although detection in Colorado may occur as soon as 2013–2014. This reduced spread in the projection is likely a trade-off between the number of caves and the length of winter ( Fig. 3 ). Species that have large geographic ranges, such as the Little Brown Bat ( M. lucifigus ), may see large population declines or extirpation at large scales [9] . Speculatively, species richness across the contiguous United States may be reduced and community structure will shift in favour of non-cave hibernating bats [30] , [31] . Predictions of spread using three climate change scenarios showed accelerated spread of WNS relative to projections based on observed data, with two caveats. First, the coarse resolution reduces the climatic variability that is consistent with mountainous regions, which coincide with the distribution of caves. Thus the projected spread rates in some regions may be reduced or accelerated by climate change in ways hard to capture with climate projections. Second, the projections had many more long winters than the observed data set, which could be due to specifics of the climate model and year-to-year variability in climate projections ( Supplementary Figs S42–44 ). As temperature appears to have a significant effect on WNS spread, actual climate, especially the amount of cold weather in the immediate future, has the potential to significantly alter rate of spread and locations infected. A potentially important puzzle piece missing from this analysis is spread within Canada. Absence of Canadian cave data (needed to estimate the cave density covariate) precluded incorporating any such infection records into our models. We suspect including such information would have decreased the estimated time to infection in Northeast counties and in the Upper Midwest, but would have had little impact on the spread into the Interior Plateaus and Highlands. It is possible that Canada could provide another route for long-distance dispersal events to reach the West. However, Canadian winters may prove to act as a barrier to dispersal because of increased mortality of bats associated with longer winters, thus limiting the number of potential dispersers. Our model is the first of which we are aware to fit WNS occurrence data to broad geographic features and identify key characteristics of spread throughout the United States. An important area for further development is construction of models representing the biological mechanisms that mediate dispersal and spread [32] . Unfortunately, key quantities such as bat-to-bat transmission probability, recovery rate, frequency of recovery, lethality and between-cave mixing at hibernacula remain unknown to us. Recent experimental evidence [7] shows that direct contact can spread the fungus from infected to uninfected bats during hibernation and that airborne exposure within artificial hibernacula does not lead to infections in susceptible individuals. Remarkably, without such a mechanistic understanding of spread, our best model matched all investigated aspects of the spatial dynamics of the epidemic, including maximum distance and number of counties infected. Although diffusive spread may occur at small scales [26] , our results show that this spread process does not scale to larger spatial extents. Our results also support an important mechanistic hypothesis: because of the relative importance of cave density in our models, we hypothesize that transmission is density-dependent at the spatial scale of infection between caves. A cave-scale proportional hazard analysis found larger colonies were more likely to have become infected, but could not distinguish between the effect of population density and the alternative that perhaps habitats preferred by bats are also more suitable for the fungus [26] . Lorch et al. [7] speculate that swarming behaviour is a likely mechanism for spread, whereby transmission between bats occurs during these fall periods of activity. As our model uses discrete time steps, it is consistent with a variety of transmission modes including the swarming hypothesis. Lorch et al. [7] provide evidence that direct exposure to conidia leads to infection within 102 days, but bat-to-bat experiments used infected bats already presenting fungal growth. It is unclear, then, if autumn swarming is indeed the dominant mechanism of transmission, as other evidence shows infection clears during the summer [33] , [34] and that the percentage of infected bats during autumn is very low [7] . We also can speculate on the effect of winter in the best-supported model. Winter length may increase transmission due to increased conidia density on surviving bats or in caves. Alternatively, longer summers may slow spread, perhaps due to increased survivorship or reduced time for the syndrome to manifest as found in infected individuals that have recovered in laboratory [34] and field settings [33] . More mechanistic models of spread, such as Susceptible-Infected-Recovered models of transmission among individual bats, could determine the importance of these effects [5] , [32] and others, such as the postulated effect of cave microclimate (humidity) on bat infection and mortality [22] , [26] . Unfortunately, data are currently too sparse to effectively estimate relevant parameters for transmission at the spatial extents considered here. Collection of individual incidence is, therefore, a priority for future empirical work [35] . Our model provides evidence for a non-diffusive spread pattern of WNS, where physical geography and environmental heterogeneity have a role in the speed and direction of spread. For other recent notable pathogens, both introduced and emergent, host ecology influences the characteristics of spread, and the combination of ecological traits exhibited by bats matches the unique mixture of heterogeneous and locally diffusive spread found here. Simulations forward suggest that spread will slow in the near future, but it will eventually reach most of the contiguous United States. Bat diversity and community structure will be affected across all of North America if the spread along the Appalachians is representative of future spread. Vespertilionid bats could be in critical danger if resistance, whether through an anthropogenic source or through evolution, does not soon emerge [9] , [10] , [36] . Data Time of infection by county was obtained from ref. 37 (ver. 1 June 2011), which records the first year of observation of WNS, presence of infectious agent G . destructans , or both. A literature search was performed to identify the number of independent infection events (that is, number of infected caves) in each county, which we refer to as ‘WNS occurrence records.’ As amplification and transmission can occur during hibernation [5] , [7] , we assigned infections to the year of first observed infection in a county where epidemic year t was assumed to begin in May t−1 and end in April t . A variable for habitat was a composite of known and estimated cave density for counties in the contiguous United States, which we consider to be a suitable proxy for the distribution of natural and anthropogenic features used by bats and suitable for G . destructans ( Supplementary Information , Supplementary Figs S45,S46 ). Average length of winter during the epidemic was estimated using the average number of days below 10 °C per year between January 2006 and December 2009, and interpolated using anisotropic ordinary kriging ( Supplementary Information , Supplementary Figs S47,S48 ). Species richness was estimated by overlaying 46 bat species range maps acquired from NatureServe ( http://www.natureserve.com ) and aggregating them by county ( Supplementary Information , Supplementary Figs S49,S50 ). Minimum daily temperature records from three climate change scenarios ( http://nomads.gfdl.noaa.gov/CM2.X/CM2.0/available_data.html ) were obtained and the length of winter was calculated for years through 2100 ( Supplementary Information ). Model Our model follows a compartmental strategy, similar to epidemiological Susceptible-Infected-Recovered models, where within-county prevalence and its potential role in spread to another county are modelled implicitly. This framework permits hypothesis testing to statistically reject potential models of spread without making assumptions regarding mechanisms determining within-county dynamics. Thus, our goal was to characterize broad geographic features that have a role in spread rather than to determine mechanisms that mediate local transmission. Our simplest hypothesis of diffusive spread without geographic complexity was investigated by fitting a model where the probability of infection between all candidate sources j and susceptible counties i declined with Euclidean distance between the centroids of i and j in an Albers equal-area projected data set of the contiguous United States through a logistic function ( Supplementary Equation S1 ). This model represents the belief that new infections are more probable in susceptible counties near infected counties. This model was modified to test for distance-decay with additional long-distance dispersal by adding a fitted parameter as an exponent of the distance between counties ( Supplementary Equation S8 ). We fit parameters of these models using all counties in the contiguous United States, followed by fitting them to a restricted number of counties defined by the presence of caves (see above). If our proxy for available hibernacula (that is, cave density) was irrelevant, then we would expect that model to fit the data equivalently or more poorly than the complete county data set. To test the hypotheses that spread was accelerated by high concentrations of caves, we fit a model that included a generalized ‘gravity’ term [38] , [39] , where the connection between counties i and j was weighted by the area of the county or density of caves in each ( Supplementary Equations S15, S20 ). This model is a generalized version of the standard gravity model in that strength of the connection was tuned by a fit parameter. This model was compared with diffusion on the restricted county network. We then tested for an effect of bat species richness by adding a term to the gravity cave model ( Supplementary Equation S21 ). Further, we tested for an effect of the number of hibernating bat species that may occur in a county during the year ( Supplementary Equation S22 ). To test the hypothesis that spread was retarded in warmer areas, we included winter duration (estimated number of days where minimum temperature was <10 °C) as a covariate ( Supplementary Equation S23 ). As climate is partially confounded with geographic position, we compared this model to one with a north–south latitudinal gradient by using the northing of the geographically projected county centroid as a covariate ( Supplementary Equation S24 ). A better fit with Supplementary Equation S23 than with Supplementary Equation S24 would indicate that temperature was the important variable, not another latitudinally varying quantity. As we found support for species richness and winter terms separately, we included both terms in a gravity model to test for improved fit ( Supplementary Equation S25 ). To allow for other forms of spread, we fit two additional dispersal kernels. First we fit a model based on Eggo et al. [19] where we modified the expression by removing a mortality term ( Supplementary Equation S26 ). The final approach was a variation on the radiation model of Simini et al. [20] in which the relationship between the cave density in two counties is weighted by the relative local population, designated as the cave density of those counties within a radius defined by the distance between the two counties ( Supplementary Equation S27 ). Changes in event probability and probability of spread associated with select models are shown in Supplementary Figs S51–53 . For each model, we created a network where each county was a node with a binary state variable representing the infected/uninfected status and edges weighted by the requisite dispersal function. ML parameters for each model were obtained using the Nelder-Mead algorithm and corroborated using a Simulated Annealing search (function optim in the R package stats [40] , Supplementary Information ). We found confidence intervals for our ML parameters using qmvnorm (package: mvtnorm [41] ) and numDeriv [42] , unless covariance matrices were not invertible ( Supplementary Information ). For a given year of spread, t +1, the probability that a given county became infected from infected counties in t for the given model and parameter set was calculated for each county. The log-likelihood of the data given the model was log-transformed binomial probability densities summed over all susceptible counties in t . The sum of log-likelihoods for each year of spread was multiplied by −1 to determine the negative log-likelihood (NLL) value for that parameter set. We compared AIC and NLL values of optimized models for model comparison. We calculated pairwise deviance explained to determine the amount of variation explained by additional parameters. To compare spatial characteristics of select model and observed data, stochastic spread was simulated from Schoharie County (time t 0 ) for 100 years ( Supplementary Information ). We repeated simulations 9,999 times and assessed county infection rate, maximum and median spread distance from Schoharie County, and area of infection. The frequency of infection and expected year of infection for each county was calculated from the full sequence of 100 winters. As this procedure ignores estimation error and misrepresents the total uncertainty associated with individual predictions, a secondary analysis was performed to propagate error due to parameter uncertainty in these models. In this analysis, 9,999 random parameter sets were obtained in proportion to the multivariate normal distribution associated with the variance-covariance matrix of the estimated parameters using the R package mvtnorm and propagated using Monte Carlo simulation (SU parameters). We then simulated spread from Schoharie County using each of 9,999 combinations of SU parameters once to assess the breadth of uncertainty in our estimated measurements. Additional simulations projected future spread from current conditions (the cumulative WNS observations as of 1 June 2011). We completed 9,999 simulations from the current observed infections and projected forward 95 winters (until 2105–2106) for both the ML and SU parameter sets. We calculated the same spread statistics as above, and examined how quickly WNS spread to regions of the country by calculating time until infection reached the maximum range of the county network, but before filling in led to saturation. Similarly, spread was simulated forward under the gravity caves +winter model using the changing winter length from the three climate change scenarios starting with 2011. Imperfect detection The preceding analyses assumed that no infected counties have gone undetected. To assess the effect of possible incomplete detection in the infection history data we simulated under-sampling using artificial data and compared results with the true (simulated) scenario without under-sampling. Infection histories were generated by simulating an ensemble of 1,000 epidemics for 5 years starting from the initial infection with the gravity caves +winter model using the ML parameter set. These infection histories constitute the true data, and from them we sampled four reduced ensembles by randomly removing 1, 5, 10, and 25% of infection records in each data set. For each of the four under-sampled ensembles we estimated the ML parameters over each infection history. This resulted in four under-sampled ensembles of 1,000 sets of model parameters, and we used each of these parameter sets to simulate an epidemic for 5 years starting from Schoharie County. For each of the four under-sampled ensembles and the one true ensemble we calculated the same spread statistics in our initial analysis. The effect of under-sampling was assessed by examining the medians and variability of the pairwise differences between the under-sampled and true spread statistics ( Supplementary Fig. S28 ). We simulated spread for 100 years with the observed climate data under the gravity caves +winter model using the 25% under-sampled data to assess the change in geographic pattern of prediction. How to cite this article: Maher, S. P. et al. Spread of WNS on a network regulated by geography and climate. Nat. Commun. 3:1306 doi: 10.1038/ncomms2301 (2012).